A highly unradiogenic lead isotopic signature revealed by volcanic rocks from the East Pacific Rise Radiogenic isotopes in oceanic basalts provide a window into the different geochemical components defining the composition of Earth’s mantle. Here we report the discovery of a novel geochemical signature in volcanic glasses sampled at a sub-kilometre scale along the East Pacific Rise between 15°37′N and 15°47′N. The most striking aspect of this signature is its unradiogenic lead ( 206 Pb/ 204 Pb=17.49, 207 Pb/ 204 Pb=15.46 and 208 Pb/ 204 Pb=36.83). In conjunction with enriched Sr, Nd and Hf signatures, Pb isotopes depict mixing lines that trend away from any known mantle end-members. We suggest that this unradiogenic lead component sampled by magmatic melts corresponds to a novel upper mantle reservoir that should be considered in the Pb isotope budget of the bulk silicate Earth. Major, trace element and isotope compositions are suggestive of an ancient and lower continental origin for this unradiogenic lead component, possibly sulphide-bearing pyroxenites that were preserved even after prolonged stirring within the ambient upper mantle. Over time, melting processes have exhausted Earth’s upper mantle of its most incompatible elements, resulting in a depleted residual reservoir (depleted mid-ocean-ridge-basalt mantle) striated by geochemical heterogeneities inherited from the recycling of contrasting ocean and continental material [1] . Basalts from mid ocean ridges (MORB) and ocean islands (OIB) are both extracted from the asthenospheric mantle, and carry within their geochemical make-up (concentrations and isotopes) the fingerprints of these ‘enriched’ re-injected materials. In particular, Sr, Pb, Nd, Hf and noble gas isotopic compositions of MORB and OIB, have been successfully used to describe the global geochemical complexity of the mantle and reduce it to a multi-component mixture of isotopic end-members [2] , [3] . Isotopic data have also demonstrated the presence of spatial mantle domains separated by geochemical boundaries, such as the Australian–Antarctic discordance [4] . On the eastern side of this limit, the Pacific upper mantle appears only enriched by subducted oceanic lithosphere, while on the other side, the Indian upper mantle is also polluted by lower continental inputs [5] . The geochemical properties of the latter, dubbed the ‘DUPAL (Dupré-Allègre) anomaly [4] , [6] ’, include lower 206 Pb/ 204 Pb, 207 Pb/ 204 Pb and 208 Pb/ 204 Pb relative to Pacific MORB. Such unradiogenic Pb signatures are unusually rare in MORB relative to expectations from global Pb isotopes mass balance of the bulk silicate Earth (BSE). Indeed, if the BSE has evolved as a closed system after core segregation, all crustal and mantle material should be equally distributed around a 4.53 Ga Geochron line in a 207 Pb/ 204 Pb versus 206 Pb/ 204 Pb diagram. However, MORB and OIB are mostly found to the right of this line; this apparent Pb paradox [7] suggests that a low U/Pb (father/daughter ratio) reservoir is hidden somewhere in the mantle. Ancient peridotites found in the Horoman orogenic massif (Japan) have recently shed light on the existence and properties of such a discrete reservoir [8] . Very low Pb isotope ratios were reported in these rocks and provide physical evidence that unradiogenic Pb could be trapped within the upper mantle as widespread and extremely refractory heterogeneous domains [8] , [9] , [10] , [11] largely untapped by basaltic melts. However, most of the MORB samples used in the global mantle geochemical scheme were dredged tens to hundreds of kilometres apart over decades of seafloor exploration. In this study, we take advantage of submersible in situ access, to adopt a sampling strategy specifically adapted to the scale of volcanic edifices and covering 15 km of a single East Pacific Rise (EPR) segment. Our results reveal the presence of an unradiogenic Pb signal never before reported for Pacific MORB and that constitutes a magmatic witness for the existence of an unradiogenic Pb upper mantle reservoir. Together with trace elements and Sr, Nd, Hf and He isotopes, these results suggest a high degree of heterogeneity below this region of the EPR, and reveal a novel MORB signature suggestive of the recycling of lower continental material (meta-gabbroic pyroxenites) into the Pacific upper mantle. Data description Here we present data from EPR on-axis basalts that display unradiogenic Pb compositions (associated with relatively enriched Sr-Nd-Hf isotopic compositions) indicative of a novel and previously cryptic upper mantle reservoir. Basaltic glasses sampled on discrete lava flows during submersible dives between 15°37′ and 15°47′N along the EPR covered a span of only 15 km, which represented one of the highest spatial resolution sampling efforts to date ( Supplementary Fig. 1 ). The data depict two sharp linear trends that are likely to reflect two binary mixtures (or pseudo-binary mixtures [12] ) and reveal the presence of high amplitude, short length-scale mantle heterogeneities in this area. While Pb isotopes are neatly correlated ( Fig. 1 ), Sr-Nd-Hf-Pb plots ( Fig. 2 ) are moderately scattered. Such dispersion in geochemical diagrams associated with mixing trends, may also be explained by non-uniformed mixing of fractional melts extracted from different sources, where depth controls the degree of homogenization [13] . 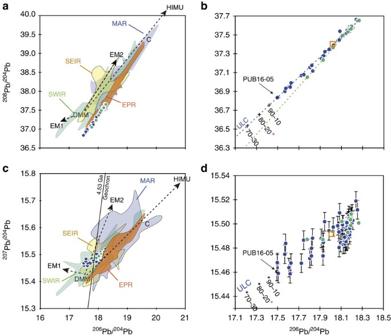Figure 1: Pb isotope compositions. Pb isotope compositions of basaltic glasses from this study (circles) and of MORB from various oceanic domains (coloured fields, SEIR: South East Indian Ridge51, SWIR: South West Indian Ridge51, MAR: Mid-Atlantic Ridge52and EPR: East Pacific Rise51). The blue and green circles in all diagrams demonstrate two different mixing trends, one between ambient mantle and unradiogenic lead component (ULC, blue circles), and one between ambient mantle and a secondary Mathematician seamount component (green circles). The mantle end-members: DMM (depleted MORB mantle), EM1 (enriched mantle type-1), EM2 (enriched mantle type-2) and HIMU (high-μ) are reported from ref.2. The common component C composition is from ref.15. (a)208Pb/204Pb versus206Pb/204Pb, (b) enlargement ofa. Both regression lines have aR2=0.99, (c)208Pb/204Pb versus206Pb/204Pb, with 4.53 Ga Geochron as reported in ref.53, (d) enlargement ofc. The black crosses correspond to theoretical compositions of the ULC component using a 70–30%, 80–20% (*preferred value) and 90−10% source mixtures for sample 10-PUB16-05 (seeSupplementary Table 2). The orange square represents the mean composition of the study samples. Error bars correspond to the external reproducibility of Pb isotope compositions (only visible on207Pb/204Pb, and smaller than the symbols for all other ratios). Figure 1: Pb isotope compositions. Pb isotope compositions of basaltic glasses from this study (circles) and of MORB from various oceanic domains (coloured fields, SEIR: South East Indian Ridge [51] , SWIR: South West Indian Ridge [51] , MAR: Mid-Atlantic Ridge [52] and EPR: East Pacific Rise [51] ). The blue and green circles in all diagrams demonstrate two different mixing trends, one between ambient mantle and unradiogenic lead component (ULC, blue circles), and one between ambient mantle and a secondary Mathematician seamount component (green circles). The mantle end-members: DMM (depleted MORB mantle), EM1 (enriched mantle type-1), EM2 (enriched mantle type-2) and HIMU (high-μ) are reported from ref. 2 . The common component C composition is from ref. 15 . ( a ) 208 Pb/ 204 Pb versus 206 Pb/ 204 Pb, ( b ) enlargement of a . Both regression lines have a R 2 =0.99, ( c ) 208 Pb/ 204 Pb versus 206 Pb/ 204 Pb, with 4.53 Ga Geochron as reported in ref. 53 , ( d ) enlargement of c . 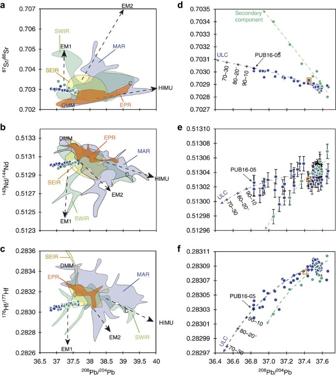Figure 2: Multiple isotope compositions. Isotope compositions of Sr (a, enlargement ind), Nd (b, enlargement ine) and Hf (c, enlargement inf) versus208Pb/204Pb. Coloured fields represent the isotopic composition of MORB from various oceanic domains (SEIR: South East Indian Ridge51, SWIR: South West Indian Ridge51, MAR: Mid-Atlantic Ridge52and EPR: East Pacific Rise51). The blue and green circles in all diagrams demonstrate two different mixing trends, one between ambient mantle and unradiogenic lead component (ULC, blue circles), and one between ambient mantle and a secondary Mathematician seamount component (green circles). The mixing trends between ambient mantle and ULC component (blue lines) can be clearly distinguished in multiple isotope spaces from the mixing trend between ambient mantle and a secondary enriched Mathematician seamount component (green lines). The mantle end-members: DMM (depleted MORB mantle), EM1 (enriched mantle type-1), EM2 (enriched mantle type-2) and HIMU (high-μ) are reported from ref.2. The common (C) component is reported from ref.15. Black crosses indicate the ULC composition assuming 90–10%, 80–20% (*preferred value) and 70–30% source mixtures for sample 10-PUB16-05 (seeSupplementary Table 2). The orange square represents the mean composition of the study samples. Error bars correspond to the external reproducibility of isotope compositions (only visible on143Nd/144Nd, and smaller than the symbols for all other ratios). The black crosses correspond to theoretical compositions of the ULC component using a 70–30%, 80–20% (*preferred value) and 90−10% source mixtures for sample 10-PUB16-05 (see Supplementary Table 2 ). The orange square represents the mean composition of the study samples. Error bars correspond to the external reproducibility of Pb isotope compositions (only visible on 207 Pb/ 204 Pb, and smaller than the symbols for all other ratios). Full size image Figure 2: Multiple isotope compositions. Isotope compositions of Sr ( a , enlargement in d ), Nd ( b , enlargement in e ) and Hf ( c , enlargement in f ) versus 208 Pb/ 204 Pb. Coloured fields represent the isotopic composition of MORB from various oceanic domains (SEIR: South East Indian Ridge [51] , SWIR: South West Indian Ridge [51] , MAR: Mid-Atlantic Ridge [52] and EPR: East Pacific Rise [51] ). The blue and green circles in all diagrams demonstrate two different mixing trends, one between ambient mantle and unradiogenic lead component (ULC, blue circles), and one between ambient mantle and a secondary Mathematician seamount component (green circles). The mixing trends between ambient mantle and ULC component (blue lines) can be clearly distinguished in multiple isotope spaces from the mixing trend between ambient mantle and a secondary enriched Mathematician seamount component (green lines). The mantle end-members: DMM (depleted MORB mantle), EM1 (enriched mantle type-1), EM2 (enriched mantle type-2) and HIMU (high-μ) are reported from ref. 2 . The common (C) component is reported from ref. 15 . Black crosses indicate the ULC composition assuming 90–10%, 80–20% (*preferred value) and 70–30% source mixtures for sample 10-PUB16-05 (see Supplementary Table 2 ). The orange square represents the mean composition of the study samples. Error bars correspond to the external reproducibility of isotope compositions (only visible on 143 Nd/ 144 Nd, and smaller than the symbols for all other ratios). Full size image One of these trends points towards very low 208 Pb/ 204 Pb and 206 Pb/ 204 Pb (36.83 and 17.49, respectively) and a moderately low 207 Pb/ 204 Pb (15.46) component that we define here as the unradiogenic lead component (ULC) ( Figs 1 and 2 ). Samples that are most imprinted by the ULC signature are located at the junction of the EPR and the Mathematician seamount chain ( Supplementary Fig. 1 ). These constitute the lowest 208 Pb/ 204 Pb and 206 Pb/ 204 Pb ratios reported for MORB from Pacific spreading centres and are among the lowest for MORB worldwide ( Fig. 1 ). Their 208 Pb/ 204 Pb and 206 Pb/ 204 Pb values overlap with those recorded on Garret EPR intra-transform lavas (13°28′S), while 207 Pb/ 204 Pb and 87 Sr/ 86 Sr are significantly higher, and Nd less radiogenic. Garrett lavas are interpreted as re-melting products of previously depleted upper mantle heterogeneity [14] . Some samples of MORB from the South West Indian ridge (SWIR) and Pitcairn Island basalts also feature similar 206 Pb/ 204 Pb and 207 Pb/ 204 Pb; however, 208 Pb/ 204 Pb ratios are higher ( Fig. 1 ; Supplementary Fig. 2 ). Abyssal peridotites can in some places display even more unradiogenic Pb compositions, but their Sr, Nd and Hf isotope signatures are always more depleted than observed for the ULC ( Supplementary Fig. 2 ). Isotopes highlight the presence of a strongly heterogeneous mantle beneath this very small portion of the ridge (0.1°), and a secondary binary mixing trend between ambient mantle and a more enriched component can also be clearly identified ( Fig. 2 ). In Sr-Nd-Hf isotope spaces, ULC-influenced basalts display enriched Indian-like MORB compositions (0.7030, 0.51303 and 0.28306, respectively), in opposition to Garrett intra-transform samples, but are otherwise unremarkable. However, together with Pb isotopes (especially the 208 Pb/ 204 Pb ratio, Fig. 2 ), these data depict an unusual trend that does not head towards any of the known ‘Mantle Zoo’ end-members [3] , [15] . Even if these trends reflected pseudo-binary mixtures, the data would still indicate the existence of a ULC capable of driving Pb isotope compositions towards unradiogenic values. Major element concentrations do not document in a straightforward way the petrological nature of ULC-basalt source, but do identify ULC-influenced melts as mostly primitive (~8% MgO). Rare earth element (REE) patterns ( Fig. 3a ) are more informative, and ULC-influenced basalt samples present patterns atypical for MORB and different from Garrett, Pitcairn and SWIR lavas. These samples feature in spidergrams ( Fig. 3 ) hump-shaped, convex patterns, slightly depleted both in light REE and heavy REE, with positive Eu, Ba and Sr anomalies, as well as Th and U depletions ( Fig. 3b ; Supplementary Fig. 3 ). 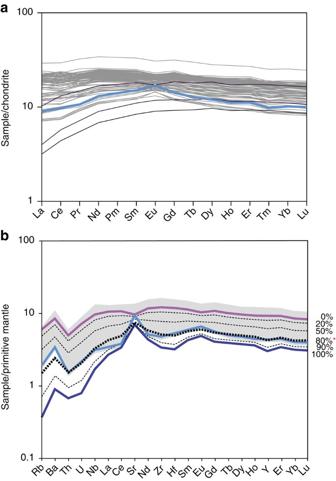Figure 3: Trace element compositions. (a) Rare Earth element compositions normalized to CI chondrite. Blue line represents the most ULC (unradiogenic lead component)-influenced sample, 10-PUB16-05. Some samples from the Garrett fracture zone are plotted as thin black lines for comparison. (b) Spider diagram of trace element mixing models normalized to the primitive Mantle54. The dark blue line corresponds to a 20% partial melt of a clinopyroxenite source. The light blue line represents the most ULC-influenced sample, 10-PUB16-05. Ambient mantle melt is represented here as a pink line and corresponds to the average composition of 40 MORB samples chosen around the intersection of the two trends inFigs 1and2. The grey field represents the whole data set. Dashed lines correspond to the result of mixing in various proportions of the metagabbroic clinopyroxenite melt with the ambient melts (seeSupplementary Table 1). The preferred values for the model (reproducing sample 10-PUB16-05, light blue line) correspond to a mixture of 4:1 metagabbroic clinopyroxenite melt with ambient melts. Figure 3: Trace element compositions. ( a ) Rare Earth element compositions normalized to CI chondrite. Blue line represents the most ULC (unradiogenic lead component)-influenced sample, 10-PUB16-05. Some samples from the Garrett fracture zone are plotted as thin black lines for comparison. ( b ) Spider diagram of trace element mixing models normalized to the primitive Mantle [54] . The dark blue line corresponds to a 20% partial melt of a clinopyroxenite source. The light blue line represents the most ULC-influenced sample, 10-PUB16-05. Ambient mantle melt is represented here as a pink line and corresponds to the average composition of 40 MORB samples chosen around the intersection of the two trends in Figs 1 and 2 . The grey field represents the whole data set. Dashed lines correspond to the result of mixing in various proportions of the metagabbroic clinopyroxenite melt with the ambient melts (see Supplementary Table 1 ). The preferred values for the model (reproducing sample 10-PUB16-05, light blue line) correspond to a mixture of 4:1 metagabbroic clinopyroxenite melt with ambient melts. Full size image The low LREE concentrations in the ULC samples are consistent with relatively high degrees of partial melting and/or very depleted sources. Moreover, the association of coinciding Eu, Sr and Ba enrichments can be directly attributed to the involvement of cumulative plagioclase in the source, a common feature of gabbros [10] , [16] and of some rare East African rift basalts [17] . This primarily gabbroic imprint on the ULC source is illustrated by Fig. 4 , where clear correlations can be observed between Pb isotopes (proxy for the ULC component) and geochemical ratios that serve as typical plagioclase markers: (CaO/Al 2 O 3 ), (Eu/Eu*) and (Sr/Eu*). The involvement of gabbroic (plagioclase cumulates) material has been previously proposed for plume melts [18] , [19] , [20] , however, plagioclase is not stable at the pressure and temperature range of mantle melting under mid ocean ridges. The material involved in this source is therefore more likely meta-gabbroic pyroxenites retaining a signature of ‘ghost plagioclase’ [20] than actual gabbros. Indeed, the hump-shaped REE patterns observed here are also common features of clinopyroxenes and pyroxenites [21] . 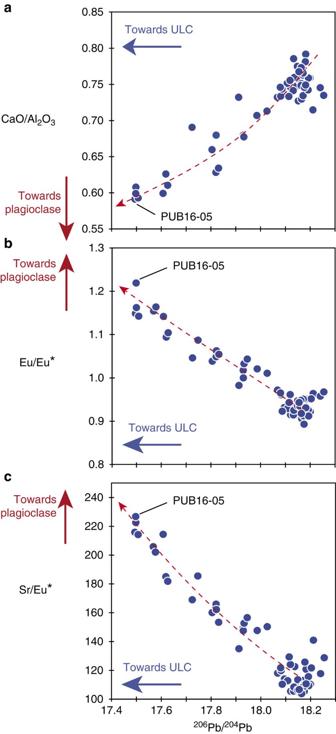Figure 4: Ghost plagioclase signature. Geochemical indicators of plagioclase involvement: (a) CaO/Al2O3, (b) Eu/Eu* and (c) Sr/Eu*, as functions of206Pb/204Pb, used here as a proxy for the unradiogenic lead component (ULC). Only samples from the ambient mantle—ULC mixing trend (blue circles and lines inFigs 1and2) are represented. All diagrams highlight the coincidence of the unradiogenic Pb signature with the geochemical imprint of ‘ghost plagioclase’. Figure 4: Ghost plagioclase signature. Geochemical indicators of plagioclase involvement: ( a ) CaO/Al 2 O 3 , ( b ) Eu/Eu* and ( c ) Sr/Eu*, as functions of 206 Pb/ 204 Pb, used here as a proxy for the unradiogenic lead component (ULC). Only samples from the ambient mantle—ULC mixing trend (blue circles and lines in Figs 1 and 2 ) are represented. All diagrams highlight the coincidence of the unradiogenic Pb signature with the geochemical imprint of ‘ghost plagioclase’. Full size image The absence of depletion in the heaviest REE (Yb and Lu) in Fig. 3 (and Supplementary Fig. 3 ) indicates that residual garnet was not present during ULC melt extraction. This is rather unexpected since, because of their alumina content, the metamorphic transformation of plagioclase cumulates into pyroxenites should involve garnet formation. The lack of a garnet signature in ULC basalts, implies that either these minerals were removed from the pyroxenites well before they entered the mantle, or more unlikely, were totally exhausted during the extraction of EPR MORB. It can be delicate to use MORB concentration data to quantitatively model partial melting processes, and thus source composition because of the complex mixing processes that occur during both melting and liquid extraction. Nevertheless, relatively simple non-modal batch melting of metagabbroic clinopyroxenites may account for the trace element signature of ULC-influenced samples. In Fig. 3b , the trace element signature of the most ULC-influenced sample (10-PUB16-05) seems to be well represented by a 1:4 mixture of peridotite melt (represented by the average of neighbouring MORB) with a melt that was extracted after 20% partial melting of pyroxenites ( Fig. 3b ; Supplementary Table 1 ). This satisfactory fit suggests that it is possible that this atypical mantle heterogeneity is largely constituted of metagabbroic pyroxenites. However, the origin of the ULC’s peculiar Pb isotope signature remains to be explained. Extrapolations of the source Pb, Hf, Nd and Sr isotope compositions are presented in Figs 1b,d and 2d–f (and Supplementary Table 2 ). Such unradiogenic Pb signatures depend on time-integrated father/daughter depletions (depressed U/Pb and Th/Pb ratios) to slow down daughter isotope production rates. The ULC reservoir must have thus been either poor in both U and Th, or significantly enriched in Pb. The second condition can be satisfied by the involvement of very large amounts of plagioclase [18] (U/Pb 0.01) or even more easily, of sulphides in which Pb is even more concentrated relative to Th and U by its chalcophilic nature. Recent investigations focused on the Re, Os and Pb isotope compositions of abyssal peridotite sulphides [11] , [22] demonstrate that the Pb isotope composition of the BSE may be largely balanced by unradiogenic Pb contained by sulphides in the mantle. However, the refractory nature of sulphide-bearing abyssal peridotites [11] , [22] render them unlikely to be involved in the source of EPR 15.4°N basalts. Furthermore, the ULC is more geochemically enriched than ultra-depleted residual peridotites [8] , [10] , [23] . Alternatively, sulphides are also common phases in ultramafic xenoliths found in the context of continental magmatic arcs [24] , [25] and may strongly influence the transfer of chalcophile elements and the composition of the sub-continental lithosphere. For example, Lee et al. [24] argue that sulphides contained in cumulative and residual continental arc roots constitute the balancing parameter of the upper continental crust’s Cu budget. Over the course of time, magmatic inflation and lithospheric shortening induce root arc thickening and the progressive burial of this material, melt fractionation, and frequently the establishment of thick metagabbroic sulphide-bearing pyroxenite roots [24] . Their high density (denser than plagioclase cumulates) makes them gravitationally unstable and they may be re-injected into the mantle, therefore contributing to the development of mantle heterogeneities [26] , [27] . Large amounts of lower crustal sulphide-bearing material may thus be continuously recycled into and sequestered in the upper mantle, and would constitute a highly unradiogenic Pb reservoir that is prone to melting. Their presence beneath EPR 15.4°N is one possible explanation for the ULC source composition. Such a scenario for the ULC requires geochemical evidence for both ancient timing and continental inheritance. The high 207 Pb/ 204 Pb ratio relative to 208 Pb/ 204 Pb and 206 Pb/ 204 Pb in the samples supports the idea that the chronometer was stopped early in Earth’s history (prior to ca. 2 Ga), when the production rate of 207 Pb was higher than those of 206 Pb and 208 Pb. Furthermore, 4 He/ 3 He ratios ( Supplementary Table 3 ) in ULC-influenced samples are systematically and significantly higher than values typical of MORB and OIB (R/Ra down to 5.6), suggesting a highly degassed source consistent with a continental inheritance [28] . The samples also display Eu/Eu*>1 and low Ce/Pb ratios that are typical of lower continental crust material [29] , [30] . While lower continental material has already been detected in the source of Indian Ocean MORB [5] , [31] , this is the first occurrence for basalts coming from a Pacific spreading centre. Furthermore, unlike these peculiar Indian Ocean MORB, ULC-influenced samples have very low 208 Pb/ 204 Pb for given 207 Pb/ 204 Pb ratios, and thus reflect a distinct geochemical signature for recycled continental material. The combination of all these geochemical properties together, therefore characterizes a source that is more compatible with re-injected fertile ultramafic cumulates (that underwent metamorphism) of continental arc root origin than with recycled lower oceanic crust. Basalts from EPR 15.4°N therefore appear to be magmatic witnesses of a fertile (compared with abyssal peridotites) and hidden Pb reservoir that, in addition to refractory peridotites, helps balance the radiogenic Pb isotope excess of the BSE. However, since its exact geochemical composition remains speculative, its actual contribution to the Pb paradox is difficult to assess. Nevertheless it is most probably minor, considering the rarity of ULC signature in MORB. The fact that this geochemical signature has never been sampled before despite decades of seafloor geochemical exploration may suggest that such material is exceptional and volumetrically insignificant within the mantle. However, a second possibility arises in the specific geodynamical setting of the EPR at 15.4°N. The ridge in this area is the shallowest and widest of the entire EPR [32] and connects to the Mathematician seamounts chain. Both the geochemical signatures of MORB and geophysical observations (thicker and more shallow seismic Axial Magma Chamber reflector [33] , ‘bulls-eyed’ negative-mantle Bouguer anomalies (MBA) [34] , [35] , two successive ridge axis jumps during the last 300 ky [33] ) strongly support ridge–hotspot interaction in this area. In this particular setting, ridge migration in the hotspot source direction is possible [36] and hotspot material is commonly assumed to be drained preferentially towards the spreading axis [37] , therefore increasing the magmatic activity of the segment. This allows its contribution to become progressively dominant in the pool melt composition. Indeed, trace element modelling suggests that to account for the trace element composition of ULC-influenced samples, hotspot melt contribution may have at times exceeded 80%. The relatively primitive nature of these basalts (~8% MgO) seems to argue for short crustal residence times, which most likely facilitate the preservation of the peculiar signature [38] . If so, it suggests that the tapping of the otherwise-silent mantle ULC signature in MORB involves the combination of several conditions: (1) abundant fertile material carrying a ULC-type signature, (2) the proximity of a hotspot and a ridge (preferential drainage of melts towards the ridge) and (3) a rapid transfer to the surface. Olivine hosted melt inclusions have already demonstrated the extraordinary geochemical variability of the mantle at very small scales [39] . The limited spatial extent (restricted to <1 km along the ridge axis) of the ULC-influenced basalt flows strongly suggests that detection of this geochemical signature was only made possible by a high-resolution (<1 m) autonomous underwater vehicle bathymetric approach that permitted high precision submersible sampling. In this study, we were able to demonstrate a MORB geochemical variability along a 15-km ridge segment that is comparable to that previously observed for the entire 9,000 km EPR. The new signature found in basaltic glasses is particularly remarkable for its highly unradiogenic Pb composition and its association with enriched Nd, Hf, Sr and degassed He isotopic signatures. Taken together, these properties indicate the recycling of ancient continental meta-gabbros. Our results strongly support the development of future petrological and geochemical studies of ocean volcanism at the same spatial scale as has been used for sub-aerial volcanism. Rock sampling Samples of basaltic glass were collected in situ with the French submersible Nautile during the PARISUB cruise (RV L’Atalante March–April 2010 (ref. 40 )). The combination of high precision bathymetric data (autonomous underwater vehicle acquisitions) and the use of the submersible allowed very accurate position determination of each sample (reported in Supplementary Table 4 and illustrated in Supplementary Fig. 1 ). Volcanic glass chips were handpicked under a microscope and ultrasonically cleaned in ultra pure milli-Q water. Data acquisition Major element concentrations were obtained using an ICP-AES Jovin Yvon Ultima 2 at the University of Brest, after a HF-HNO 3 digestion as described in ref. 41 . Trace element concentrations were measured with a Thermo Element2 HR-ICP-MS in Brest, after a repeated HF-HClO 4 digestion, and HNO3 dilutions (see ref. 42 for details). The repeated analysis of the international standard BCR2 demonstrated an external reproducibility better than 5–10% depending on the element and concentration ( Supplementary Table 5 ). Pb, Hf, Sr and Nd isotope compositions were obtained from single HF-HNO 3 dissolutions of 500 mg–1 g of sample following the protocol described by ref. 43 for Hf, Nd and Pb. Sr was separated from the Nd fraction using Eichrom Sr-specific resin following the protocol of ref. 44 adapted from ref. 45 . Pb, Hf and some of the Nd (* in Supplementary Table 3 ) isotopes were analysed using the Thermo Neptune MC-ICP-MS of Ifremer-Brest. Sr and the rest of Nd isotopes were obtained using a Thermo Triton TIMS at the University of Brest. 2σ internal errors for Hf, Nd and Sr are reported in Supplementary Table 3 and never exceeded the last significant digit (1E-5) in each analysis. Values used for mass bias fractionation corrections were 205 Tl/ 203 Tl=2.388; 88 Sr/ 86 Sr=8.375202; 146 Nd/ 144 Nd=0.7219 and 179 Hf/ 177 Hf=0.7325, for Pb, Sr, Nd and Hf, respectively. Measured values were compared with international standards: NBS981 (ref. 46 ): 208 Pb/ 204 Pb=36.7007, 207 Pb/ 204 Pb=15.4891, 206 Pb/ 204 Pb=16.9656; JMC475 (ref. 47 ): 176 Hf/ 177 Hf=0.282157); La Jolla [48] : 143 Nd/ 144 Nd=0.511858; JNDI [48] : 143 Nd/ 144 Nd=0.512115; and NIST987: 86 Sr/ 87 Sr=0.710248. He isotopes were obtained using a noble gas mass spectrometer Nu Noblesse at the Institute de Physique du Globe de Paris following the protocol presented in Moreira et al . [9] All results are reported in Supplementary Table 3 (isotopes), Supplementary Table 6 (major elements) and Supplementary Table 7 (trace elements). Trace element modelling We used a simple non-modal batch melting model [50] combined with liquid–liquid mixing to testify that the partial melting of a meta-gabbroic clinopyroxenite and subsequent mixing with basaltic melts can generate trace element patterns similar to ULC samples. Where C L represents concentration in the melt, C 0 the initial source rock concentrations, D and P the bulk partition coefficients and F the degree of partial melting. Global D and P were calculated for a metagabbroic clinopyroxenite constituted of 80% Cpx and 20% Opx and using elemental partition coefficients (Kd) from a combination of several references from the literature reported in Supplementary Table 1 . The trace element compositions used for this source is HR-10 gabbro [10] ( Supplementary Table 1 ), because of its similar trace element pattern and its unradiogenic Pb. LREE element depletion of ULC-influenced basalts, and pyroxenite being more fertile than peridotite, both suggest a high degree of partial melting. We thus decided to set it arbitrarily at 20%. Ambient mantle melt compositions were estimated by averaging 40 sample compositions, picked around the intersection of the blue and green trends of Figs 1 and 2 . All the modelling parameters are summarized in Supplementary Table 1 and results of the calculations are reported in Fig. 3b . The model suggests that 80–20% mixture of the metagabbroic pyroxenite melt and ambient mantle melt, respectively, can convincingly reproduce the most extreme ULC-influenced sample (10-PUB16-05) composition. The model also indicates that the ULC fingerprint on trace elements patterns disappears when the amount of pyroxenite melts in the mixture is <50%. Isotope modelling A simple isotope-mixing model has been applied. The basic assumption is that the blue trend of Figs 1 and 2 represents the binary mixture between clinopyroxenite (ULC) melt of unknown isotope composition and an average ambient mantle melt whose isotope compositions correspond to the intersection of the blue and green trends in Figs 1 and 2 . The proportions considered for the ULC melt in 10-PUB16-05 (the extreme end-member of the blue trend) are those obtained based on the trace element modelling: 80% ULC melt+20% ambient mantle melt. Because this estimation is speculative, we also considered neighbouring ranges of composition (70–30 and 90–10) for comparison. All parameters and results are reported in Supplementary Table 2 and the modelled compositions for ULC are represented in Figs 1 and 2 . How to cite this article: Mougel, B. et al. A highly unradiogenic lead isotopic signature revealed by volcanic rocks from the East Pacific Rise. Nat. Commun. 5:4474 doi: 10.1038/ncomms5474 (2014).